Valley spin polarization by using the extraordinary Rashba effect on silicon The addition of the valley degree of freedom to a two-dimensional spin-polarized electronic system provides the opportunity to multiply the functionality of next-generation devices. So far, however, such devices have not been realized due to the difficulty to polarize the valleys, which is an indispensable step to activate this degree of freedom. Here we show the formation of 100% spin-polarized valleys by a simple and easy way using the Rashba effect on a system with C 3 symmetry. This polarization, which is much higher than those in ordinary Rashba systems, results in the valleys acting as filters that can suppress the backscattering of spin-charge. The present system is formed on a silicon substrate, and therefore opens a new avenue towards the realization of silicon spintronic devices with high efficiency. Spintronic devices [1] , [2] , [3] , [4] , [5] , [6] , [7] , a new scheme of electronics using the spin degrees of freedom together with the electron charge, can be classified into two categories, the magnetic spintronic devices for information storage, and semiconductor ones such as the spin field-effect transistor [1] for logical operations. Of these two categories, the realization of semiconductor spintronic devices is far behind the magnetic ones, which already appear in the market as, for example, read heads of hard disk drives. The main reason is the difficulty to handle the spin current, the key principle for operating semiconductor spintronic devices. In nonmagnetic materials, spin degeneracy is lifted by spin–orbit coupling in combination with space inversion asymmetry, such as at solid surfaces and interfaces, that is, the so-called Rashba effect [8] , [9] . Ordinarily, the Rashba effect produces a pair of spin-polarized bands in k space with the spin polarization vector in the surface plane and a Fermi surface consisting of two concentric circles with opposite chiral spin textures. As shown in Fig. 1a , the presence of these two Fermi circles allows electrons to backscatter, and thus can greatly reduce the efficiency of the spin transport. Topological insulators with a single Dirac cone [10] , a new state of matter, show a single circle with chiral spin texture ( Fig. 1b ) that would prevent backscattering of electrons in the opposite direction provided the spin is 100% polarized and there is no influence of magnetic impurities. However, owing to the actual spin polarization that is far from 100% (ref.11) [11] and the tilting of the spin direction [12] , electron spins can be backscattered in this material as well [13] . Consequently, the complete suppression of backscattering, an essential requirement to achieve high performance semiconductor spintronic devices [13] , is still an unresolved issue. In this respect, a very promising approach is combining valley physics, which restricts the scattering direction as in the case of graphene [14] , [15] ( Fig. 1c ), with two-dimensional spin-polarized electronic systems. It is also crucial to spin-polarize the valleys, as shown in Fig. 1d , which provides the filtering function that suppresses the probability of backscattering. Furthermore, previous propositions for valley polarization in graphene require difficult ways of electron confinement. In contrast, we propose a simple and easy method. 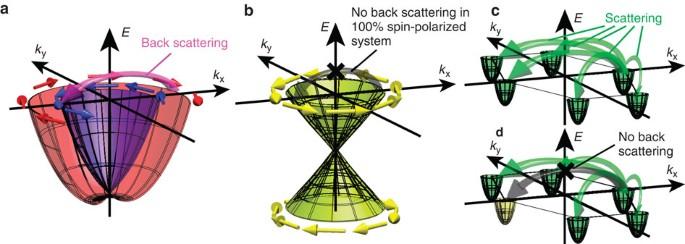Figure 1: Dispersion and spin texture of spin-polarized bands and the valley scattering. Spin-polarized bands of (a) an ordinary Rashba system and (b) topological insulator. (c) A system with non-polarized electron valleys at theandpoints of the SBZ. In this case, scattering is limited to the—() directions, which is in contrast to the case of systems with Fermi circles at thepoint where electrons scatter in all directions. (d) A system in which one valley, the one indicated by yellow, is polarized. Electrons cannot backscatter in this case. Figure 1: Dispersion and spin texture of spin-polarized bands and the valley scattering. Spin-polarized bands of ( a ) an ordinary Rashba system and ( b ) topological insulator. ( c ) A system with non-polarized electron valleys at the and points of the SBZ. In this case, scattering is limited to the — ( ) directions, which is in contrast to the case of systems with Fermi circles at the point where electrons scatter in all directions. ( d ) A system in which one valley, the one indicated by yellow, is polarized. Electrons cannot backscatter in this case. Full size image Here, we show that a Si(111) surface with slightly more than one monolayer (ML) of Tl on top forms 100% spin-polarized valley surface states for which the backscattering can be tuned to disappear. The heavy element Tl gives rise to the strong spin–orbit coupling, which induces the large spin splitting responsible for the spin-polarized valleys, and the use of Si as substrate will issue a guideline to the realization of silicon spintronic devices [16] , [17] , [18] . The atomic structure of the Tl/Si(111)-(1 × 1) surface at a coverage of 1 ML and the corresponding surface Brillouin zone (SBZ) are displayed in Fig. 2a . Tl atoms are adsorbed on the 3-fold hollow site (the T 4 site) of a Si(111)-(1 × 1) ideal surface, leading to a 3-fold symmetric structure with mirror planes in the [ ] and the two other corresponding directions. This surface structure leads to the (and ) points to have C 3 symmetry, which lifts the spin degeneracy at these points and forces the polarization vector of the fully polarized spin to be perpendicular to the surface [19] , [20] , [21] . This differs from that of normal Rashba systems, where the polarization is parallel to the surface and perpendicular to the wave vector ( Fig. 1a ). The out-of-plane spins of the occupied surface state, which were observed experimentally with high-resolution angle-resolved photoelectron spectroscopy (ARPES) [20] and discussed theoretically [19] , [21] , are unfortunately far below the Fermi level and will therefore hardly contribute to any charge transport. 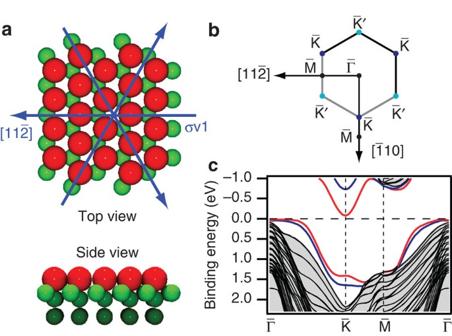Figure 2: Basic properties of Tl/Si(111)-(1×1). (a) Atomic structure of the system. Red and green circles represent the Tl and Si atoms, respectively, and the blue arrows indicate the mirror planes. (b) The SBZ of Tl/Si(111)-(1 × 1). The symmetry pointsandare indicated by dark-blue and light-blue circles. (c) Energy-band dispersions obtained by a relativistic first-principles band calculation. Red and blue lines are spin-polarized surface states. Figure 2: Basic properties of Tl/Si(111)-(1 × 1). ( a ) Atomic structure of the system. Red and green circles represent the Tl and Si atoms, respectively, and the blue arrows indicate the mirror planes. ( b ) The SBZ of Tl/Si(111)-(1 × 1). The symmetry points and are indicated by dark-blue and light-blue circles. ( c ) Energy-band dispersions obtained by a relativistic first-principles band calculation. Red and blue lines are spin-polarized surface states. Full size image Electronic structure of undoped Tl/Si(111) As displayed in Fig. 2c , theoretical calculations predict the presence of an unoccupied surface electronic band with a substantially larger spin splitting just above the Fermi level at the point. This suggests a possibility to make a metallic spin-polarized band by doping electrons into the Tl/Si(111)-(1 × 1) surface while keeping the substrate semiconducting as there are no bulk continuum states at the corresponding energies. In Fig. 3a , we show the occupied electronic band of an undoped Tl/Si(111)-(1 × 1) surface obtained by ARPES and the unoccupied band obtained by spin- and angle-resolved inverse photoemission spectroscopy (SARIPES) along the k x direction in Fig. 3b . The Rashba splitting is clearly observed in the occupied state, and two spin-polarized surface bands are observed above the Fermi level. The polarization vectors of these unoccupied surface bands are perpendicular to the surface and the spins are 100% polarized as in the case of the occupied states at the point. This experimental finding agrees well with the polarization vector predicted in the theoretical calculation. 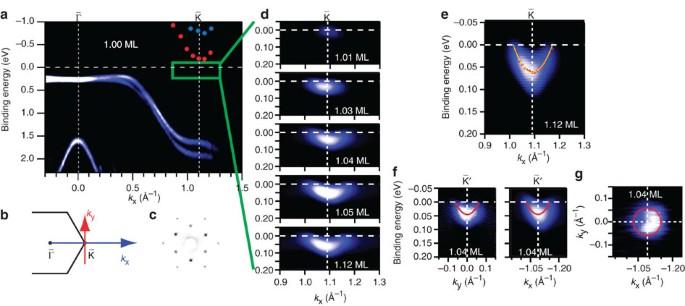Figure 3: Spin-polarized metallic band. (a) ARPES result together with the SARIPES one, which is indicated by red and blue circles of a Si(111) surface covered with 1.00 ML of Tl. (b) Directions ofkxandkywith respect to the SBZ. (c) Low-energy electron diffraction pattern of the Tl/Si(111)-(1 × 1) surface obtained at a Tl coverage of 1.00 ML with a primary electron energy of 111 eV. (d) Metallic band observed at thepoint for different Tl coverages. The area indcorresponds to the area indicated by the green box ina. Detailed band dispersion of the metallic band at a Tl coverages of (e) 1.12 ML along thekxdirection and (f) of 1.04 ML along thekxandkydirections. (g) Fermi surface of Si(111) covered with 1.04 ML of Tl. Figure 3: Spin-polarized metallic band. ( a ) ARPES result together with the SARIPES one, which is indicated by red and blue circles of a Si(111) surface covered with 1.00 ML of Tl. ( b ) Directions of k x and k y with respect to the SBZ. ( c ) Low-energy electron diffraction pattern of the Tl/Si(111)-(1 × 1) surface obtained at a Tl coverage of 1.00 ML with a primary electron energy of 111 eV. ( d ) Metallic band observed at the point for different Tl coverages. The area in d corresponds to the area indicated by the green box in a . Detailed band dispersion of the metallic band at a Tl coverages of ( e ) 1.12 ML along the k x direction and ( f ) of 1.04 ML along the k x and k y directions. ( g ) Fermi surface of Si(111) covered with 1.04 ML of Tl. Full size image Electronic structure of doped Tl/Si(111) In this study, we doped the Tl/Si(111)-(1 × 1) surface by adsorbing a small amount of extra Tl. The extra Tl does not change the low-energy electron diffraction pattern for Tl coverage of 1.00–1.12 ML ( Fig. 3c ). As shown in Fig. 3d , a state appears at the Fermi level with an extra Tl coverage of 0.01 ML, and it moves continuously downward in energy by adding more and more Tl. This agrees with the appearance of a metallic property with extra Tl in former studies [22] , [23] . This result demonstrates that electrons are doped into the unoccupied surface state. To quantitatively discuss the observed metallic band obtained at Tl coverages of 1.12 and 1.04 ML, we show close ups of the band in Fig. 3e and f , respectively. The red dots in Fig. 3e mark the peak positions of the metallic band extracted from the ARPES spectra, and the yellow line represents the dispersion obtained by fitting the peak positions using a parabola. The result indicates that the bottom of the metallic band is located at a binding energy ( E B ) of 65 meV, and that the effective mass is ~0.35 m e along the k x direction at 1.12 ML. At 1.04 ML, the bottom of the metallic band is shifted to E B =45 meV, but the effective mass is the same. This agrees with a rigid-shift picture of the spin-polarized unoccupied surface band by electron doping. Furthermore, in the light of the same effective mass along the k y direction and the roughly circular shape of the Fermi surface shown in Fig. 3g , we conclude that the spin-polarized metallic band of the Tl/Si(111)-(1 × 1) surface forms valleys with a parabolic shape at the and points. Spin-polarized valleys To grasp the overall character of the metallic band, the spin-resolved ARPES (SARPES) spectra measured around the and points along the k y direction, and those around the point along the k x direction are shown in Fig. 4a for a sample with Tl coverage of 1.12 ML. Here, the SARPES spectra were obtained with an experimental setup that is sensitive to spins with polarization vectors perpendicular to the surface ( z direction). The red and blue spectra represent the spin pointing in the positive (spin-up) and the negative z direction (spin-down) as shown in the inset. It is apparent from these spectra that the metallic band is 100% spin-up at the point, and 100% spin-down at the point. The correspondence between the spin directions of the metallic band and those of the occupied bands located at an E B of about 2 eV agrees well with the spin directions predicted theoretically ( Fig. 2c ). The time-reversal symmetry [ E ( k ,↑)= E (− k ,↓)] is preserved in this system, but the inversion asymmetry lifts the spin degeneracy and leads to opposite spin directions at and . Therefore, the metallic valleys are polarized intrinsically in this peculiar Rashba system. 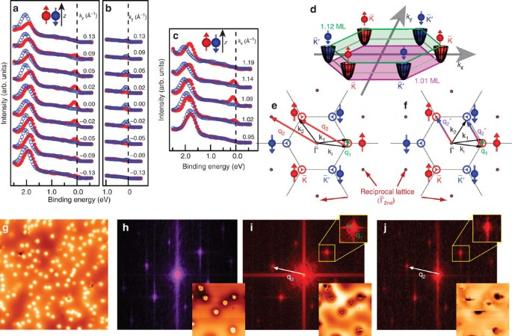Figure 4: Spin character of the metallic band. SARPES spectra measured along thekydirection around (a) thepoint and (b) thepoint, and (c) along thekxdirection around thepoint. The directions of the wave vectorskxandkyare shown inFigure 3b. The red (blue) spectra represent the spin pointing to positive (negative)zas indicated in the inset. (d) Schematic illustration of the spin-polarized surface states atand. The green (purple) hexagon represents the SBZ. The position of the SBZ is here used to indicate the Fermi level at a coverage of 1.12 (1.01) ML. Illustrations of scattering processes (e) without and (f) with spin flipping.kiis the wave vector of the incident electrons, andk1andk2are the wave vectors of the scattered ones.q1andq2(q2′) are the intravalley and intervalley scattering wave vectors. (g) A 41.7 × 41.7 nm2STM image of a Si(111) surface with 1.01 ML of adsorbed Tl.Vsampleand tunneling current are +1.0 V and 3.0 nA, respectively. (h) Two-dimensional FFT map of an STM topography obtained for a sample with <0.0005 ML of extra Tl at aVsampleof +0.25 V. The inset inhis the 30 × 30 nm2STM topography.qspace maps of scattering amplitudes obtained from FFT ofdI/dVmaps atVsampleof (i) +0.5 V and (j) +0.25 V. The insets iniandjare the quasiparticle interference patterns of 30 × 30 nm2images. Figure 4: Spin character of the metallic band. SARPES spectra measured along the k y direction around ( a ) the point and ( b ) the point, and ( c ) along the k x direction around the point. The directions of the wave vectors k x and k y are shown in Figure 3b . The red (blue) spectra represent the spin pointing to positive (negative) z as indicated in the inset. ( d ) Schematic illustration of the spin-polarized surface states at and . The green (purple) hexagon represents the SBZ. The position of the SBZ is here used to indicate the Fermi level at a coverage of 1.12 (1.01) ML. Illustrations of scattering processes ( e ) without and ( f ) with spin flipping. k i is the wave vector of the incident electrons, and k 1 and k 2 are the wave vectors of the scattered ones. q 1 and q 2 ( q 2 ′ ) are the intravalley and intervalley scattering wave vectors. ( g ) A 41.7 × 41.7 nm 2 STM image of a Si(111) surface with 1.01 ML of adsorbed Tl. V sample and tunneling current are +1.0 V and 3.0 nA, respectively. ( h ) Two-dimensional FFT map of an STM topography obtained for a sample with <0.0005 ML of extra Tl at a V sample of +0.25 V. The inset in h is the 30 × 30 nm 2 STM topography. q space maps of scattering amplitudes obtained from FFT of dI/dV maps at V sample of ( i ) +0.5 V and ( j ) +0.25 V. The insets in i and j are the quasiparticle interference patterns of 30 × 30 nm 2 images. Full size image Figure 4d shows schematically the spin-resolved electronic structure of a Si(111) surface with slightly more than 1 ML of Tl on top. The green (purple) hexagon represents the SBZ, here drawn to indicate the position of the Fermi level with a Tl coverage of 1.12 (1.01) ML. The Fermi level of the 1.12 ML Tl surface cuts through the parabolic metallic band, resulting in constant-energy contours at the Fermi level (the Fermi surface) as small circles with a radius of ~0.1 Å −1 centred at the and points. This Fermi surface resembles closely that of an electron-doped graphene single layer [24] , although the underlying dispersions and the spin properties are different. The graphene single layer is associated with a pseudo spin instead of real spin. Scattering process The Fermi surface and its spin structure govern the elastic electron scattering between states located in a single valley (intravalley scattering), and states located in two valleys at ( ) points or one at and the other at (intervalley scattering). k i in Fig. 4e denotes the wave vector of the incident state, and k 1 and k 2 are the wave vectors of the scattered states. Of the two dominant classes of scattering vectors, q 1 corresponds to intravalley scattering, and q 2 ( q 2 ′ ) to intervalley scattering between two points or two points (between and ). The absence of intervalley scattering between and in Fig. 4e results from the fact that the spin at the valley is completely opposite to that at the valley so that the overlap of the scattered wave to the incident one is zero if the spin-flip does not occur as in Fig. 4f . This is different from the graphene case in which the intervalley scattering between and occurs due to the helical pseudo spin texture [25] , [26] , [27] . To confirm the scattering process experimentally, we performed a scanning tunnelling microscope (STM) study of Tl/Si(111)-(1 × 1) surfaces with extra Tl. Figure 4g shows a 41.7 × 41.7 nm 2 topographic STM image of a surface with 0.01 ML of extra Tl. As shown in this figure, the apparent size of the extra Tl adsorbates (bright spots in the image) has a diameter of ~1.3 nm that makes it difficult to observe the electronic structure of the bare Tl/Si(111)-(1 × 1) surface area. Thus, the study of the quasiparticle interference pattern, which is indispensable to understand the scattering process, was not possible at the smallest coverage showing a metallic band in ARPES. We therefore decreased the amount of extra Tl to <0.0005 ML and accessed the electron scattering at unoccupied states above the Fermi level. The rigid-shift model of the spin-polarized unoccupied surface band allows us to discuss the scattering process under this condition. Figure 4h displays a reciprocal lattice map obtained by a two-dimensional fast Fourier transform of an STM topography image of the sample with <0.0005 ML of extra Tl. The six reciprocal lattice points located in the second Brillouin zones are clearly observed together with weak signals from reciprocal lattice points of the third Brillouin zones. (Note that the hexagon formed by the six reciprocal lattice points in Fig. 4h appears rotated compared with those shown in Fig. 4e . The orientation of the hexagons in Fig. 4h just reflects the actual orientation of the sample in the STM set up.) Quasiparticle interference patterns are observed in the dI/dV mapping obtained at V sample =+0.5 V and +0.25 V (inset of Fig. 4i ). The q space maps of scattering amplitudes obtained from fast Fourier transform of these dI/dV maps are displayed in Fig. 4i . The bright spots in these figures appear at exactly the same position as those of the reciprocal lattice points. At V sample =+0.5 V, which corresponds to an energy of 0.25 eV above the bottom of the valley, both the intravalley scattering vectors q 1 and the intervalley one q 2 are observed. Of these two vectors, the length of q 1 , ~2.7 nm −1 , agrees well with the diameter of the valley obtained experimentally by SARIPES and by theoretical calculations at the corresponding energy. As extra spots located at the ( ) positions (the positions of the and points) should appear in the case of spin-flip scattering just like the spots observed in graphene due to the scattering vector q 2 ′ [25] , [26] , [27] (refs25–27), the results in Fig. 4i indicate that there is no spin-flip scattering in the present case. As shown in Fig. 4i , scattering in the diametrically opposite direction via q 2 is restricted but scattering might occur via q 1 , and thus the backscattering probability is restrained but not zero at V sample =+0.5 V. At V sample =+0.25 V, that is, the scattering at the bottom of the valley, q 1 becomes infinitely small and only q 2 remains. As the spin polarization vector remains unchanged at the bottom of the valley, this indicates the absence of any scattering in the diametrically opposite direction. Note that in contrast to the present case, backscattering would be possible even at the bottom of the valley in normal Rashba systems with spin polarization parallel to the surface. The present study shows that the Rashba effect on a system with C 3 symmetry completely spin polarizes the valleys in an easy and simple way and makes them acting as filters that suppress the backscattering of spin carriers. Thus, combining peculiar Rashba spins with valleytronics opens up an avenue to greatly improve the efficiency of spin currents for silicon spintronics applications. Sample preparation method A Si(111) surface was cleaned by annealing up to 1,520 K for a few seconds. Tl was deposited onto the clean Si surface at 300 K, followed by annealing at 500 K for a couple of minutes. The intensity of the Tl 5d core level was monitored to obtain the Tl coverage. ARPES measurements All PES experiments were performed in ultrahigh vacuum chambers under a base pressure of <5 × 10 −9 Pa. High-resolution ARPES and SARPES measurements have been carried out at different laboratories. ARPES data have been obtained at synchrotron radiation facilities, beamline I4 at MAX-lab, Sweden and the APE beamline at Elettra, Italy, using photon energies from 15 to 40 eV, with energy and momentum resolutions of 10 meV and below 1% of the SBZ, respectively. The sample was maintained at 100 K during the ARPES measurements. The SARPES experiments were performed at beamline 19 A at Photon Factory, High Energy Accelerator Research Organization, Japan, using a photon energy of 17 eV at an energy resolution of 20 meV and momentum resolution below 2% of the SBZ. A very-low-energy-electron-diffraction-type spin polarimeter [28] was part of the data collection system. SARIPES measurements The experiments were performed at the University of Münster, Germany, in an ultrahigh vacuum apparatus (base pressure <3 × 10 −9 Pa) with a combined SARIPES and SARPES setup [29] . The SARIPES data were retrieved by using spin-polarized electrons with energy between 7 and 14 eV emitted from a GaAs photocathode and detecting photons from the sample with a Geiger-Müller counter at a detection energy of 9.9 eV. STM measurements The STM experiments were performed in an ultrahigh vacuum cryogenic STM (Unisoku, Japan), equipped with a Nanonis controller (Specs, Germany). The base pressure was 6 × 10 −9 Pa, and the temperature was maintained at 78 K. The topography and dI/dV maps were simultaneously taken by a lock-in detection method with a modulation voltage of 10–20 mV at 1–2 kHz and a set point of 0.1–3 nA. Density functional theory calculation Calculations were carried out by using the generalized gradient approximation [30] in the Kohn-Sham theory [31] . The energy cutoffs of 25 and 300 Ry were used for wave functions and charge densities [32] , and a repeated slab model was used for the surface calculation. The slab contains a Tl ML, 24 Si ML and 1 H ML. The atomic positions, except those of the H atoms and the Si atoms bonded to H, were fully optimized to an assumed criterion of atomic force (<0.01 eV Å −1 ). The slabs were separated by 9.7 Å of vacuum. How to cite this article: Sakamoto, K. et al . Valley spin polarization by using the extraordinary Rashba effect on silicon. Nat. Commun. 4:2073 doi: 10.1038/ncomms3073 (2013).